miRNAs confer phenotypic robustness to gene networks by suppressing biological noise miRNAs are small non-coding RNAs able to modulate target gene expression. It has been postulated that miRNAs confer robustness to biological processes, but clear experimental evidence is still missing. Here, using a synthetic biological approach, we demonstrate that microRNAs provide phenotypic robustness to transcriptional regulatory networks by buffering fluctuations in protein levels. We construct a network motif in mammalian cells exhibiting a ‘toggle-switch’ phenotype in which two alternative protein expression levels define its ON and OFF states. The motif consists of an inducible transcription factor that self-regulates its own transcription and that of a miRNA against the transcription factor itself. We confirm, using mathematical modelling and experimental approaches, that the microRNA confers robustness to the toggle-switch by enabling the cell to maintain and transmit its state. When absent, a dramatic increase in protein noise level occurs, causing the cell to randomly switch between the two states. MicroRNAs (miRNAs) are small non-coding RNAs able to modulate protein expression by pairing to cognate sites at the 3′-untraslated region of target mRNAs, thus promoting mRNA degradation and/or translation inhibition. The role of miRNAs is still under debate because, unlike transcription factors, the phenotype induced by their perturbation (that is, knockdown or overexpression) is usually subtle [1] . For example, in Caenorhabditis elegans , systematic knockout of single miRNA, or even double or triple mutants, fails to elicit an observable phenotype [2] , [3] , [4] . It has been postulated that miRNAs have a pivotal role in conferring robustness to biological processes against enviromental fluctuations during development [5] , [6] , [7] and, more generally, in buffering fluctuations in gene expression [1] , [5] , [6] , [7] , [8] , [9] , [10] , [11] , [12] , [13] . Biological robustness has been defined as the ability to correctly perform a biological function against endogenous and exogenous perturbations [14] , such as stochastic fluctuations in gene expression. This ‘biological noise’ has long been observed in both prokaryotes and eukaryotes, where it increases phenotypic variability among individual cells [15] , [16] , [17] , [18] . Increased cell-to-cell variability has been found to be either benificial, such as during stress or differentiation, or detrimental such as during embryonic development of multicellular organisms, where it can decrease robustness if not properly controlled [19] . For example, correct development of sensory organs in Drosophila depends on the presence of the miRNA miR-7, but only in the face of environmental perturbations [5] . Indeed, miR-7-mutant animals subjected to fluctuating environmental temperature fail to form complete antennae, whereas wild-type larvae develop normally [5] . So far, the ability to elucidate the role of miRNAs in conferring robustness to a biological process has been hampered by the difficulty in clearly distinguishing the contribution of the miRNA from the crosstalk of all the other regulatory pathways that control the same biological process. Indeed, miRNA-mediated negative feedback loops (NFLs) are often found coupled to multiple transcriptional feedback loops in gene regulatory networks across species and collaborate with transcription factors (TFs) to regulate their targets [5] , [13] , [20] . Synthetic biology can be used to assess, in a controlled setting, the contribution of the miRNA to the overall phenotype exhibited by an engineered biological circuit [12] , [21] . This is a complementary approach to the investigation of miRNAs in an endogenous setting and it can uncover the design principles underlying biological robustness. We construct a simple but non-trivial network motif (positive NFL—PNFL) exhibiting a ‘toggle-switch’ phenotype created by two alternative protein expression levels (ON and OFF). The motif consists of a TF that regulates its own transcription (positive feedback loop—PFL) and that of a naturally occurring human miRNA directed against the TF itself (miRNA-mediated NFL). The main phenotype of a toggle-switch is the ability to maintain an ON (high protein level) or OFF (low protein level) state indefinitely across multiple cell divisions and to switch only when a specific signal is transiently applied. Mathematical and experimental analyses demonstrate that the PNFL motif is a robust toggle-switch, whereas the motif lacking the miRNA (that is, the PFL motif) is not. Indeed, the PFL motif will spontaneously switch ON because of a higher noise level, thus clearly demonstrating the role of miRNAs in conferring phenotypic robustness to transcriptional networks. A synthetic PNFL network motif We constructed a PNFL motif in Chinese Hamster Ovary (CHO) made up of well-known and characterized biological parts, orthogonal to the endogenous ones, assembled as depicted in Fig. 1 . 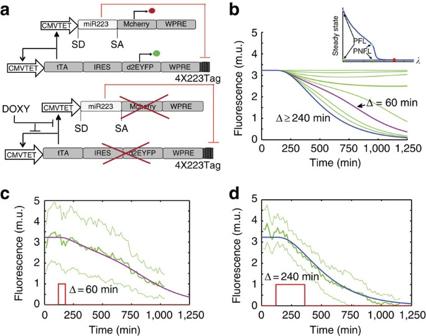Figure 1: Schematics of the PNFL motif and ‘switch-OFF’ experiments following pulses of doxycycline of different duration. (a) The tetracycline-controlled transactivator (tTA) is self-regulated, in the absence of doxycycline, by binding the tTA-responsiveCMV-TETpromoter, thus generating a PFL (black lines), whose dynamics is tracked by a destabilized EYFP (d2EYFP). The sameCMV-TETpromoter drives the transcription of the human miRNA miR-223 embedded in the first intron of the low-affinity nerve growth factor receptor (ΔLNGFR)23, followed by a reporter gene encoding for the mCherry fluorescent protein (NFL—red lines). miR-223 in turn downregulates the tTA mRNA levels through four-repeated target sequences perfectly complementary to the miR-223 seed sequence, placed at the 3′-untraslated region of the PFL gene expression cassette. Doxycycline interrupts the tTA-mediated transcriptional activation. WPRE, woodchuck hepatitis virus post-transcription regulatory element. (b) Simulated d2EYFP fluorescence of PNFL cells following simulated treatment with doxycycline of different duration Δ. In the inset, the bifurcation diagram when varying the miRNA strength (λ) is shown. (c,d) Experimental d2EYFP fluorescence using the microfluidics device (solid green line) following treatment with doxycycline (red line) at time 120 min and removal after Δ=60 min (c) or 240 min (d); s.d. is among at least three replicates (thin green lines); simulations (blue and purple lines) are rescaled to the experimental data and also represented inb(same colours). Figure 1: Schematics of the PNFL motif and ‘switch-OFF’ experiments following pulses of doxycycline of different duration. ( a ) The tetracycline-controlled transactivator (tTA) is self-regulated, in the absence of doxycycline, by binding the tTA-responsive CMV-TET promoter, thus generating a PFL (black lines), whose dynamics is tracked by a destabilized EYFP (d2EYFP). The same CMV-TET promoter drives the transcription of the human miRNA miR-223 embedded in the first intron of the low-affinity nerve growth factor receptor (ΔLNGFR) [23] , followed by a reporter gene encoding for the mCherry fluorescent protein (NFL—red lines). miR-223 in turn downregulates the tTA mRNA levels through four-repeated target sequences perfectly complementary to the miR-223 seed sequence, placed at the 3′-untraslated region of the PFL gene expression cassette. Doxycycline interrupts the tTA-mediated transcriptional activation. WPRE, woodchuck hepatitis virus post-transcription regulatory element. ( b ) Simulated d2EYFP fluorescence of PNFL cells following simulated treatment with doxycycline of different duration Δ. In the inset, the bifurcation diagram when varying the miRNA strength ( λ ) is shown. ( c , d ) Experimental d2EYFP fluorescence using the microfluidics device (solid green line) following treatment with doxycycline (red line) at time 120 min and removal after Δ=60 min ( c ) or 240 min ( d ); s.d. is among at least three replicates (thin green lines); simulations (blue and purple lines) are rescaled to the experimental data and also represented in b (same colours). Full size image The PNFL motif consists of a synthetic TF (tetracycline-responsive transcriptional activator; tTA) binding its own promoter (CMV-TET), thus self-activating its own expression. The binding of the TF to the promoter can be inihibited by doxycycline. The TF also binds another promoter (CMV-TET) driving expression of a naturally occuring mammalian miRNA (miR-223). miR-223 is specifically expressed in the myeloid lineage, where it targets multiple genes inducing a low magnitude of repression, mainly acting as a rheostat to adjust protein output [22] . The miRNA, once expressed, targets the mRNA encoding for the TF, thanks to four sequence tags at the 3′-end of the transcript perfectly complementraty to the miR-223 seed sequence [23] (see Supplementary Note 1 ). We embedded the positive feedback motif and negative feedback motif in two separate lentiviral vectors; we then performed sequential integration in CHO cells. The ability of lentiviruses to randomly integrate in the genome of the host cells, with different expression levels of the transgene according to the site of integration, allowed us to generate nine monoclonal populations of CHO cells (PFL cells) carrying the PFL motif shown in Fig. 2a . PFL clones were then used to generate 14 matched PNFL clonal populations of CHO cells (PNFL cells), carrying both PFL and the NFL cassettes shown in Fig. 1a (see also Supplementary Figs S1 and S2 and Supplementary Note 2 ). 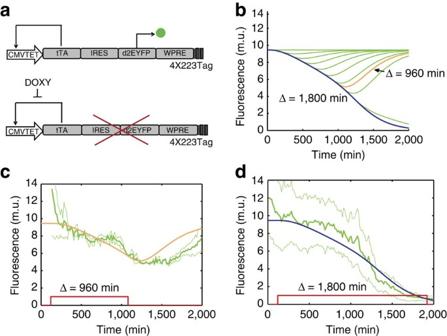Figure 2: Schematics of the PFL motif and ‘switch-OFF’ experiments following pulses of doxycycline of different duration. (a) The tetracycline-controlled transactivator (tTA) is self-regulated, in the absence of doxycycline, by binding the tTA-responsiveCMV-TETpromoter, thus generating a PFL (black lines), whose dynamics is tracked by a destabilized EYFP (d2EYFP). (b) Simulated d2EYFP fluorescence of PFL cells following simulated treatment with doxycycline of different duration Δ. (c,d) Experimental d2EYFP fluorescence using the microfluidics device (solid green line) following treatment with doxycycline (red line) at time 120 min and removed after Δ=960 min (c) or 1,800 min (d); s.d. (thin green lines) is among at least three replicates; simulations (blue and orange lines) are rescaled to experimental data and also represented inb(same colours). Figure 2: Schematics of the PFL motif and ‘switch-OFF’ experiments following pulses of doxycycline of different duration. ( a ) The tetracycline-controlled transactivator (tTA) is self-regulated, in the absence of doxycycline, by binding the tTA-responsive CMV-TET promoter, thus generating a PFL (black lines), whose dynamics is tracked by a destabilized EYFP (d2EYFP). ( b ) Simulated d2EYFP fluorescence of PFL cells following simulated treatment with doxycycline of different duration Δ. ( c , d ) Experimental d2EYFP fluorescence using the microfluidics device (solid green line) following treatment with doxycycline (red line) at time 120 min and removed after Δ=960 min ( c ) or 1,800 min ( d ); s.d. (thin green lines) is among at least three replicates; simulations (blue and orange lines) are rescaled to experimental data and also represented in b (same colours). Full size image Dynamic behaviour of the PNFL network motif To examine the dynamic behaviour of the PNFL motif, we developed a mathematical model of eight nonlinear differential equations (for details refer to Supplementary Note 3 ). This model is an extension of a model we previously published for the PFL motif to which we added four extra equations describing the miR-223 and the mCherry protein [24] . The extra parameters, specific to the PNFL model, were chosen to minimize the error between model predictions and experimental observations ( Supplementary Fig. S3 and Supplementary Table S1 ). The PNFL model consists of the following ordinary differential equations: where T m =tTA mRNA, T p =tTA protein, M i =inactive form of the miRNA, M a =active form of the miRNA. The first equation represents the transcription rate of the tTA mRNA ( T m ) as the sum of a production term, proportional to a function f ( T p , D) of the tTA protein level ( T p ) and of doxycycline (D), and a degradation term, proportional to the mRNA degradation rate ( d 1 ) plus the effect of the miRNA ( λ · g ( M a )). The parameter λ represents the strength of the miRNA. By setting λ =0, the effect of the miRNA is abolished, thus obtaining the model of the PFL motif, as described by equations (1) and (2). The second equation describes the protein translation rate of the tTA protein as proportional to the amount of mRNA ( T m ) and to the protein degradation rate ( d 2 ). The third and fourth equations describe the transcription rate of the miRNA from the tTA inducible promoter and its maturation. Specifically, in the third equation, the transcription rate of the miRNA ( M i ) is proportional to a production term, G 2 f ( T p , D), which is a function of the tTA protein T p binding to the miRNA promoter, and to a degradation ( d 3 ) plus maturation ( K D ) term. The fourth equation describes the maturation rate of the mature miRNA ( M a ) as a function of the immature miRNA and of the degradation rate of the mature miRNA. For simplicity, we omitted four additional linear differential equations that are needed to model the translantion and maturation of the two fluorescent reporters ( Supplementary Note 3 for the full model). We explored the behaviour of the PNFL motif and its robustness to model parameters by numerical bifurcation analysis. As shown in the inset of Fig. 1b and in Supplementary Fig. S4 , the PNFL can behave as a bistable system (toggle-switch), which, in the absence of doxycycline, can either be ON (high expression of the d2EYFP) or OFF (low expression of the d2EYFP) as long as the repression of the miRNA is not too strong. Specifically, when the level of the TF is above the promoter activation threshold, the PFL motif will switch ON and stay ON because of its autocatalytic activity; if, however, the TF activity is transiently blocked (that is, by a small molecule or signalling event), then its protein product will decrease below the promoter activation threshold and the PFL will switch OFF and stay OFF even after the transient block has been removed [11] , [24] , [25] , [26] , [27] , [28] . To explore the dynamic properties of the PNFL motif, we simulated in silico a series of ‘switch-OFF’ experiments. The switch-OFF simulations were performed starting from the ON steady-state and then simulating treatment with doxycycline for a limited time interval (Δ). Numerical simulations of the d2EYFP fluorescence level in Fig. 1b for the PNFL model, and in Fig. 2b for the PFL model (used as a control) show that, in both cases, when the duration of doxycycline treatment is below a threshold value ( min and min), d2EYFP expression initially decreases (switches OFF) and then increases back ON once doxycycline is removed. However, when the doxycycline treatment lasts longer than the threshold duration Δ th , d2EYFP expression switches OFF and it does not increase again, even after doxycycline has been removed. This is the telltale feature of a bistable ‘toggle-switch’. To experimentally probe the toggle-switch behaviour of the PNFL circuit, and to confirm numerical simulations, we used an innovative microfluidics platform coupled to an inverted epifluorescence microscope to administer doxycycline and to follow in real time d2EYFP fluorescence in clonal populations of PFL and PNFL cells [29] ( Supplementary Notes 4 and 5 for details on the microfluidic device). We selected a clonal population of PFL cells (PFL-7 in Supplementary Fig. S2 ) and a matched clonal population of PNFL cells (PNFL 7–2 in Supplementary Fig. S2 ) derived from the same PFL clone. We then performed in vitro ‘switch-OFF’ experiments by treating PNFL and PFL cells with doxycycline (at a concentration of 1 μ g ml −1 ) for a limited time interval (Δ). The duration Δ of doxycycline treatments was chosen according to the in silico analysis performed with the PNFL and PFL models. d2EYFP fluorescence measurements ( Fig. 1c,d for the PNFL circuit, and Fig. 2c,d for the PFL) confirmed the results of the in silico analysis, showing that the PNFL is bistable: indeed, treatment with a pulse of doxycycline lasting 60 min ( Fig. 1c ) or 240 min ( Fig. 1d ) permanently switched the circuit OFF, whereas a pulse of 20 min did not cause any visible effect ( Supplementary Fig. S5 ). The PFL had the same overall behaviour but its dynamics were much slower ( Fig. 2c,d ). Moreover, as detailed in the next section, we further probed the bistable behaviour of additional PFL and PNFL clones by fluorescent-activated cell sorter (FACS), as reported in Fig. 3 and Supplementary Fig. S6 . 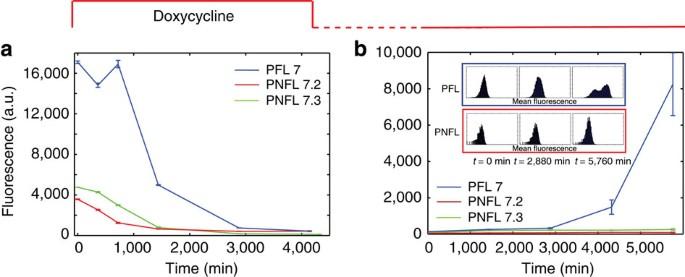Figure 3: FACS switch-OFF experiment of PFL and PNFL cells. (a) d2EYFP fluorescence levels in PFL cells (blue line) and PNFL 7–2 and 7–3 cells (red and green line, respectively) were measured at 0, 6 (360 min), 12 (720 min), 24 (1,440 min), 48 (2,880 min) and 72 h (4320, min) following treatment with doxycycline (1 μg ml−1) at time 0 h. (b) d2EYFP fluorescence levels in PFL cells (blue line) and PNFL cells (red line) cells were measured at 0, 24 (1,440 min), 48 (2,880 min) and 96 h (5,760 min) following the removal of doxycycline at time 0 h. Before time 0 h, both PFL and PNFL cells were grown in the presence of doxycycline for 72 h. (Subpanel): histogram displaying FACS data for PFL-7 (blue frame) and PNFL 7–2 (red frame) at timest=0, 2,880 and 5,760 min; CVs computed at 0, 24, 48 and 72 h are, respectively, 74.5, 105.1, 108 and 202.6 for PFL and 81.9, 88.4, 85.75 and 96 for the PNFL, thus revealing the higher variability for PFL clones compared with PFL. Error bars represent the s.d. among three replicates. Figure 3: FACS switch-OFF experiment of PFL and PNFL cells. ( a ) d2EYFP fluorescence levels in PFL cells (blue line) and PNFL 7–2 and 7–3 cells (red and green line, respectively) were measured at 0, 6 (360 min), 12 (720 min), 24 (1,440 min), 48 (2,880 min) and 72 h (4320, min) following treatment with doxycycline (1 μg ml −1 ) at time 0 h. ( b ) d2EYFP fluorescence levels in PFL cells (blue line) and PNFL cells (red line) cells were measured at 0, 24 (1,440 min), 48 (2,880 min) and 96 h (5,760 min) following the removal of doxycycline at time 0 h. Before time 0 h, both PFL and PNFL cells were grown in the presence of doxycycline for 72 h. (Subpanel): histogram displaying FACS data for PFL-7 (blue frame) and PNFL 7–2 (red frame) at times t =0, 2,880 and 5,760 min; CVs computed at 0, 24, 48 and 72 h are, respectively, 74.5, 105.1, 108 and 202.6 for PFL and 81.9, 88.4, 85.75 and 96 for the PNFL, thus revealing the higher variability for PFL clones compared with PFL. Error bars represent the s.d. among three replicates. Full size image miRNA confers phenotypic robustness by buffering noise Ideally, once the toggle-switch is OFF, it should stay OFF indefinitely. However, because of the autocatalytic nature of both PFL and PNFL motifs (that is, a TF self-activating its own promoter), it should be much easier for both motifs to stay ON than to stay OFF. Indeed, when the switch is OFF, small fluctuations in the TF protein levels may be amplified by the PFL, causing the system to switch back ON [16] . To analyse the effect of the miRNA on noise propagation in the PNFL network motif, we considered a simplified stochastic gene expression model with transcription, translation and degradation as probabilistic events occurring at exponentially distributed time intervals [30] , [31] ( Supplementary Fig. S7 ). Specifically, in the model, mRNAs are produced in transcriptional bursts from the promoter, in agreement with the recent modelling and experimental evidences concerning noise in eukaryotic gene expression [15] , [16] , [32] . We then derived, under a set of simplifying assumptions ( Supplementary Note 6 ), a system of differential equations describing the dynamics of the statistical moments in four different scenarios ( Supplementary Fig. S7 and Supplementary Table S2 ): (1) unregulated transcription, that is, the mRNA is transcribed from a constitutive promoter [30] ; (2) regulated transcription where the protein activates its own transcription (that is, the PFL motif); (3) a NFL mediated by the miRNA inducing degradation of the target mRNA (that is, a NFL motif); (4) the PNFL motif when both PFL and the miRNA-mediated NFL are present (Methods and Supplementary Note 6 ). Finally, we computed an analytical expression for the coefficient of variation (CV), that is, the relative deviation of protein expression in each cell compared with the population average, which can be used as a measure of noise. Indeed, a small CV corresponds to a tight distribution centred around the mean, hence a small cell-to-cell variability; a large CV corresponds to a loose distribution, indicating large cell-to-cell variability. From the analytical expression of the CV in the four scenarios ( Supplementary Note 6 ), it can be deduced that, independently of the model parameter values, noise increseas when a transcriptional PFL is present, compared with unregulated transcription, in agreement with previous modelling and experimental results [15] , [16] , [27] . On the contrary, noise decreases, compared with unregulated transcripiton, when a miRNA-mediated NFL is present, again in agreement with previous modelling and experimental results on negative feedbacks [15] , [16] , [33] . In the case of the PNFL motif, when both negative and positive feedbacks are present, noise is reduced compared with the PFL motif, but is greater than the unregulated transcription. To investigate the validity of the stochastic model predicitions, we measured the distribution of fluorescence levels across the cells in each of the monoclonal cell populations (9 for the PFL and 14 for the PNFL) as shown in Fig. 4a . We then quantified the protein noise level by computing the CV as the relative deviation of d2EYFP fluorescence in each cell compared with the clonal population average. 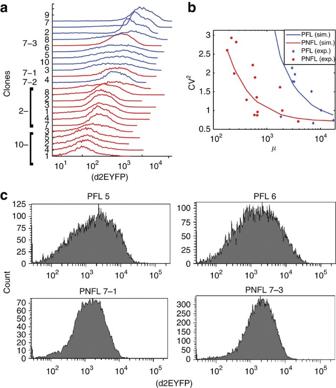Figure 4: The miRNA-mediated NFL reduces fluctuations in protein expression. (a) FACS-derived histograms of the distribution of d2EYFP fluorescence for the 9 clonal populations of PFL cells (in blue) and the 14 clonal populations of PNFL cells (in red). (b) Experimental (dots) and simulated (solid lines) values of CV2as a function of mean fluorescence for PFL clones (in blue) and PNFL clones (in red); the simulated CV2values were computed as described inSupplementary Note(equations (10)–(19)). (c) FACS-derived histograms of the distribution of d2EYFP fluorescence in two representative clonal populations of PFL and PNFL cells with similar average fluorescent intensities (PFL 5,6 and PNFL 7–1, 7–3). Figure 4b reports the theoretical CVs derived for both PFL and the PNFL stochastic models, superimposed to the experimentally measured CVs in the 23 clones (9 PFL and 14 PNFL; see also Supplementary Note 7 and Supplementary Fig. S8 and Supplementary Table S3 ). Figure 4: The miRNA-mediated NFL reduces fluctuations in protein expression. ( a ) FACS-derived histograms of the distribution of d2EYFP fluorescence for the 9 clonal populations of PFL cells (in blue) and the 14 clonal populations of PNFL cells (in red). ( b ) Experimental (dots) and simulated (solid lines) values of CV 2 as a function of mean fluorescence for PFL clones (in blue) and PNFL clones (in red); the simulated CV 2 values were computed as described in Supplementary Note (equations (10)–(19)). ( c ) FACS-derived histograms of the distribution of d2EYFP fluorescence in two representative clonal populations of PFL and PNFL cells with similar average fluorescent intensities (PFL 5,6 and PNFL 7–1, 7–3). Full size image Figure 4c shows representative examples of the d2EYFP fluorescence distribution of two PFL clones and two PNFL clones, with similar average fluorescence intensities; Fig. 4b shows the CV for all the PFL and PNFL clones. The experimental results clearly demonstrate a reduced protein noise level (CV) in the PNFL cells as compared with the PFL cells, indicating a specific effect of the miRNA-mediated negative feedback in buffering protein expression fluctuations. The PFL motif is predicted to have a higher noise level than the PNFL motif because fluctuations in the number of transcribed mRNAs are translated into fluctuations in the number of proteins, which in turn control the number of transcribed mRNAs. This results in a net amplification of noise ( Supplementary Note 7 ). On the other hand, when the miRNA-mediated negative feedback is present, noise is reduced because fluctuations in the number of mRNA molecules amplified by the PFL are counterbalanced by the presence of the miRNA. We decided to evaluate the phenotypic robustness of both PNFL and PFL motifs in terms of how long they were able to stay OFF in the absence of doxycycline. We performed a long-term experiment by treating monoclonal population of PNFL cells and their matched control population of PFL cells with doxycycline for 72 h (4,320 min); we then washed doxycycline out and monitored d2EYFP fluorescence in cells for 96 h (5,760 min) by FACS. If both motifs exhibit a robust phenotype, then they should not re-express d2EYFP and stay permanently OFF. As shown in Fig. 3a , for the PFL-7 clone and the matched PNFL 7–2 and 7–3 clones, following doxycycline treatment, both PNFL and PFL cells switched d2EYFP expression OFF, with dynamics similar to those estimated using the microfluidics set-up. Strikingly, following doxycycline washout, PFL cells started switching back ON at 72 h (4,320 min) and fully expressed d2EYFP at 96 h (5,670 min; Fig. 3b ). On the contrary, PNFL cells stayed OFF ( Fig. 3b ). As further confirmation of the miRNA role, we performed the same experiment on PNFL cells but this time inhibiting the action of the miRNA by transfection with a locked nucleic acid complementary to the miR-223 sequence (LNA 223) [34] . PNFL cells treated with the LNA increased d2YFP expression at 72 and 96 h, whereas PNFL cells treated with a control LNA maintained their OFF state, confirming our previous results (details and data are shown in Supplementary Note 8 and Supplementary Fig. S9 ). We repeated the long-term experiment on additional PFL and matched PNFL clones to exclude that the difference in phenotypic robustness we observed was clone specific. As reported in Supplementary Fig. S6a,b for the PFL-2 and PNFL 2–2, 2–3 and 2–7 clones, and in Supplementary Fig. S6c,d for the PFL-10 and PNFL 10–2 clones, the presence of the miRNA-mediated feedback loop consistently confers robustness to the PFL motif, allowing the PNFL cells to maintain their OFF state for longer as compared with the matched PFL cells. The main difference among the three PFL clones (PFL7, PFL2 and PFL10) was observed in the time taken to switch back ON following doxycycline removal ( Fig. 3b and Supplementary Fig. S6b,d ). This difference is probably because of the different insertion site of the PFL cassette in the genome of the three clones. The combination of computational analysis coupled with experimental biology, at the core of synthetic biology, has been used as a powerful tool to elucidate complex cellular processes, such as cell polarization [35] and transcriptional regulation [12] . Here we used the synthetic biology paradigm to explore the role of miRNAs in conferring robustness to a fundamental network motif, the PFL. A PFL enables a gene regulatory network to encode a ‘cellular memory’ because of its switch-like behaviour created by two different stable states [36] , [37] . Transitions across the states (that is, switching) can be triggered by a specific endogenous or exogenous event [8] , [11] , thus enabling the control of key decision processes such as cell differentiation and cell fate in response to specific clues [38] . The switch-like behaviour of the PFL motif, however, comes at a cost: first, the PFL may considerably slow down the transcriptional response of the circuit to the triggering event [24] ; this can be acceptable, or necessary, in some cases, but detrimental in others; the second and biggest issue is that the PFL motif increases biological noise because small fluctuations in the expression levels of the TF are amplified by the self-regulatory loop. The increased cell-to-cell variability in the TF concentration may cause the TF level to be higher than the promoter activation threshold, inducing transition of the switch from the OFF state to the ON state, even in the absence of the triggering event [8] , [36] . Here we experimentally demonstrated that the presence of a miRNA suffices to solve both issues at once, by conferring phenotypic robustness to the toggle-switch, thanks to the reduction of biological noise, and by enabling the circuit to respond faster. Therefore, the difference in robustness between the PNFL and PFL motifs can be explained by taking into account the ‘stochastic switching’ phenomenon. Stochastic fluctuations in gene expression, because of biological noise, will induce random transitions between the two states of the toggle-switch [36] , [39] , [40] . Interestingly, if the miRNA repression on the target mRNA is too strong, then the PNFL will no longer be able to function as a toggle-switch because of a loss of bistability ( Supplementary Fig. S4 ). This intuitively means that the miRNA will force the circuit to always be OFF by inhibiting the TF expression. In addition, the stronger the miRNA repression, the smaller the difference between the OFF state and the ON state in terms of protein expression levels. These constraints may have contributed to the evolution of the weak transcriptional effect exerted by the majority of the known miRNAs. A recent experimental and computational analysis investigated the properties of the incoherent feedforward loop motif consisting a TF inducing expression of both a reporter gene and a miRNA directed against the same reporter gene [12] . The authors demonstrated that the feedforward loop motif made the reporter gene expression level insensitive to the motif-carrying plasmid copy-number. Moreover, they observed that the presence of the miRNA led to a reduced variability in reporter protein expression among cells transfected with the motif-carrying plasmid. Deans et al . [41] used a small short-hairpin RNA to enhance the robustness and performance of an inducible mammalian genetic switch. Our results add further support to the role of miRNAs as noise suppressor. In addition, we demonstrated that reducing noise is essential to maintain a robust phenotype by preventing cells from unwanted stochastic switching. We believe that our findings on the role of the miRNA explain the abundance of miRNA-mediated negative feedbacks in gene regulatory networks across species [13] , [20] . Indeed, it was previously suggested [13] that miRNA-mediated NFLs may be needed to reduce intracellular noise, thus conferring phenotypic robustness to the pathways they are part of. Here we demonstrated that indeed this is the case. One of the best studied examples of PNFL in vivo is the E2F1/miR-17-92 network [13] , [42] , [43] . Here the E2F1 TF, a main regulator of cell cycle, regulates its own transcription and that of the miR-17-92 cluster targeting E2F1 itself. According to our results, and as previously suggested, the role of the miRNA-mediated NFL should be of preventing stochastic activation of E2F1 leading to unwanted proliferation or apoptosis [13] , [43] . In addition, several developmental TFs are regulated by PFLs [38] . These PFLs could be frequently coupled to miRNA-mediated NFLs to prevent untimely activation of the TF, which would probably be lethal for the developing embryo [13] . For example, the muscle regulatory factor MYOD activates its own transcription [44] , [45] as well as transcription of miRNAs predicted to target MyoD itself [43] , [46] . Another example is provided by intestinal cell specification in the nematode C . elegans during embryonic development. This process is regulated by a PFL involving elt-2 , the master regulatory gene of intestinal differentiation [19] . Raj et al . [19] demonstrated that stochastic activation of the elt-2 PFL underlies incomplete penetrance of mutant embryos, leading to pronounced phenotpyic variability. A limitation of our synthetic network approach is that the miRNA seed sequence is perfectly complementary to the four recognition sites we engineered at the 3′- ttA_IRES_d2EYFP of the mRNA ( Fig. 1a ). A perfectly complementary-binding site causes the miRNA to induce a catalytic-like RNA interference process, rather than the more subtle gene expression ‘thresholding’ effect observed in endogenous miRNA-binding sites [47] . This effect causes the miRNA-induced target mRNA repression to decrease, and eventually be completely abolished, if the target mRNA increases above a certain threshold saturating the miRNA pool [47] . Our results are relevant to endogenous miRNA regulation as long as the mRNA expression remains below the threshold, as, in this situation, endogeneous miRNA-binding sites and perfectly complementary-binding sites have very similar effects [47] . Our findings are a direct proof of the essential role of miRNAs in providing phenotypic robustness to a biological process. Our results are also relevant to the growing field of synthetic biology, in that they demonstrate how to synthetize robust circuits by employing miRNA-mediated feedback loops. Construction of PNFL network in CHO cells The synthetic circuit was implemented in a lentiviral vector using the ViraPower Promoterless Lentiviral Gateway Expression System (Invitrogen). The pMAtTA-IRES-EGFP-WPRE vector was synthesized by GENEART. The d2EYFP encoding gene from pd2EYFP-1 (Clontech) was substituted in place of the EGFP to generate a new vector termed pMAtTA-IRES-d2EYFP. The pMAtTA-IRES-d2EYFP was recombined with the pDONR221 (Invitrogen) to yield the pENTRtTA-IRES-d2EYFP vector. The pMA-miR-223-destRFP-WPRE vector [48] was synthesized by GENEART. An mCherry fluorescent protein-encoding gene was substituted for the RFP to generate the pMA-miR-223-mCherry-WPRE. The CMV-TET promoter was amplified from pTRE2 (Clontech) using PCR and inserted into a pENTR5′-TOPO vector to obtain the pENTR5′-TOPO- CMV-TET with specific recombination sites. We performed recombination reactions between the pENTRtTA-IRES-d2EYFP/pENTR-miR-223-mCherry, pENTR5′-T OPO- CMV-TET and the pLenti/R4R2/V5-DEST according to manufacturer’s instructions. Cell culture and clone generation CHO cells were maintained at 37 °C in a 5% CO2-humidified incubator and cultured in α-MEM (Sigma) supplemented with 10% heat-inactivated fetal bovine serum (Invitrogen), 1% L -glutamine and 1% antibiotic/antimycotic solution (GIBCO BRL). To transduce cells with the virus produced, 500,000 CHO cells were plated and incubated overnight. On the day of transduction, the medium was removed and 1 ml of the virus was added to the cells together with polybrene (Invitrogen) to a final concentration of 6 μg ml −1 . After an overnight incubation, the medium containing the virus was removed and replaced with complete culture medium containing blasticidin (Sigma) to a final concentration of to select for stably transduced cells. Cells were sorted for fluorescence intensity using a BD FACSAria Cell Sorting System (Becton Dickinson). d2EYFP was excited at 488 nm, and emission was detected using a 525-nm bandpass filter. Serial dilutions of stably transduced cells (up to 0.05 cells per ml) were plated in 96-well microtitre plates, and dilutions containing only one cell per well were selected. Monoclonal colonies were cultured and amplified as described, to obtain monoclonal populations [24] . Monoclonal CHO-PFL cell lines were transduced with the virus carrying the NFL with the same procedure. Monoclonal population of infected cells were isolated as described above to generate the PNFL cell lines. Fluorescence-activated cell sorting Cells from 35 mm culture plates were trypsinised, filtered and subjected to FACS analysis in a Becton Dickinson FACSAria, using excitation and emission filters described above. Each phenotypical analysis was performed in biological duplicates. Switch-OFF and switch-ON experiments PFL-7 and PNFL 7.2 cells were plated in a 12-well culture plate to obtain 400,000 cells per well, and then treated (or mock-treated) with 1 μg ml −1 doxycycline. Fluorescence was measured by FACS analysis at 0, 6, 12, 24, 48 and 72 h after treatment. The doxycycline-containing medium was replaced 48 h after treatment. For the switch-ON experiments, PFL-7 and PNFL 7.2 cells were pretreated with 1 μg ml −1 doxycycline for 72 h and then plated as described above, either in medium containing doxycycline or not (control). Fluorescence was measured by FACS at 0, 24, 48, 72 and 96 h after treatment. For both switch-OFF and switch-ON experiments, each FACS measurement was made on a sample of 20,000 events in duplicate. Microfluidics and microscopy We used the microfluidic device for mammalian cell culture described in ref. 49 . Before cell loading, the channels in the device were coated with 100 μg ml −1 fibronectin for 1 h at room temperature. After coating, the fibronectin solution was removed using a vacuum manifold, and a high density cell suspension (10 7 cells per ml) was loaded in the dedicated inlet. PFL and PNFL cells were loaded into the cell traps at a seeding density of 10–20 cells per trap, and the device was placed in a cell culture incubator to allow attachment of cells. The device was then placed under a Nikon Eclipse TI-E inverted epifluorescence microscope, equipped with an incubation chamber (H201-OP R2, Okolab). The two syringes connected to the inlets were filled with untreated medium or medium containing 1 μg ml −1 doxycycline. Sulforhodamine 101 (Sigma-Aldrich, Germany), a fluorescent dye, at a concentration of 1 μM was added to the medium containing doxycycline. The flow was adjusted to provide doxycycline for a given time interval (40, 60 and 180 min for PNFL cells and 960 or 1,800 min for PFL cells). Bright-field and fluorescence images of 3–20 traps per experiment were acquired with a × 40 objective at intervals of 15 min. Fluorescence images were taken using fluorescein isothiocyanate (for d2EYFP, excitation 460/40 nm and emission 510/50 nm) and tetramethylrhodamine isothiocyanate (for sulforhodamine 101: excitation 530/30 nm and emission 590/60 nm) filters. Images were acquired using a Peltier-cooled Andor Clara camera controlled by Nikon Instrument Software AR v.3.22.14. Image acquisition and processing was performed as described in ref. 24 ( Supplementary Note 9 ). Dynamical model of the PNFL To model the behaviour of the PNFL motif, we develop a mathematical model of eight nonlinear ordinary differential equations (ODEs) as detailed in Supplementary Note 3 . Numerical simulations were run using Matlab 2010b (Mathworks Inc.). For the parameter identification, we used the PottersWheel toolbox [50] implemented in MATLAB, which is also described in ref. 24 . Stochastic models of the PFL and PNFL circuits Following a stochastic model of gene expression [30] , we derived the squared coefficient of variation CV 2 =( σ / μ ) 2 for the PFL and PNFL circuits, as well as of a control circuit without any feedback non-positive feedback loop (NOPFL), as described in Supplementary Notes 6 and 7 . How to cite this article: Siciliano, V. et al . miRNAs confer phenotypic robustness to gene networks by suppressing biological noise. Nat. Commun. 4:2364 doi: 10.1038/ncomms3364 (2013).